Design and discovery of a novel half-Heusler transparent hole conductor made of all-metallic heavy elements Transparent conductors combine two generally contradictory physical properties, but there are numerous applications where both functionalities are crucial. Previous searches focused on doping wide-gap metal oxides. Focusing instead on the family of 18 valence electron ternary ABX compounds that consist of elements A, B and X in 1:1:1 stoichiometry, we search theoretically for electronic structures that simultaneously lead to optical transparency while accommodating intrinsic defect structures that produce uncompensated free holes. This leads to the prediction of a stable, never before synthesized TaIrGe compound made of all-metal heavy atom compound. Laboratory synthesis then found it to be stable in the predicted crystal structure and p -type transparent conductor with a strong optical absorption peak at 3.36 eV and remarkably high hole mobility of 2,730 cm 2 V −1 s −1 at room temperature. This methodology opens the way to future searches of transparent conductors in unexpected chemical groups. Transparent conductors (TCs) needed in solar cell, light emitting diode and flat panel displays [1] , [2] , [3] , [4] , [5] , represent the usually contraindicated functionalities of optical transparency (generally associated with electrical insulators) coexisting with electrical conductivity (generally associated with optically opaque metals) [6] . The search of TCs has generally focused on chemical groups characterized as light element wide gap oxides, such as Al-doped ZnO [7] , (for n -type) or CuAlO 2 [8] , and K-doped SrCu 2 O 2 [9] (for p -type) TCs. Rather than attempting discovery within such a preconceived chemical neighbourhood (either by high-throughput computation [10] or via combinatorial synthesis), the discovery of TCs might be guided instead by a set of physics-based metrics that p -type TCs need to satisfy a priori [9] , [11] , [12] , [13] , [14] then search not only light element oxides or nitrides but allow for a broader range of chemistries to be inspected. Such ‘Design Principles’ include a combination of (a) electronic structure features of the perfect crystal and, in parallel, (b) properties of the non-stoichiometric defected lattice. In category (a) we require a wide (>2.5 eV) direct band gap for optical transparency (but the non-absorbing indirect band gap can be significantly smaller), whereas good mobility requires rather light (<0.5 m 0 ) hole effective mass and a bulk hole wavefunction that avoids as much as possible the close neighbourhood of the ions so as to minimize scattering. In category (b) we require that the intrinsic defects are hole producers (acceptors such as cation vacancies), have low formation enthalpy (that is, be abundant) and have shallow acceptor levels (that is, be readily ionizeable), whereas the intrinsic defects that are ‘hole killers’ (donors such as anion vacancies) must have high formation enthalpy. In considering such design principles it is not obvious a priori that only the traditionally sought light element oxides are eligible for satisfying these simultaneous conditions. We choose to focus on the 18-electron ABX compounds that represent diverse chemical groups such as A n B 10 X (8− n ) as well as A ( n +1) B 9 X (8− n ) ( n =1, 2, 3, 4) with atoms spanning columns 1–5, 9–17 in the Periodic Table. This broad range of atoms (albeit within the group of ABX) encompasses a broad range of chemistries including light as well as heavy elements; anions as well as cations. The previously synthesized members from these groups manifest extraordinary functionalities such as thermoelectricity, superconductivity, piezoelectricity and topological insulation, but as yet no TCs. But not all atom combinations that, by the current understanding of solid-state chemistry, can plausibly lead to such ABX structures are in fact realized. For example, from a total of 483 possible 18 valence electron ABX compounds from the above noted chemical groups, only 83 are known [15] , whereas 400 are, in fact, ‘missing compounds’ that might constitute an attractive playing ground for new materials with new functionalities. We [16] , [17] and others [18] , [19] have developed theoretical, first principles techniques for examining the thermodynamic stability of missing compounds sorting out the ‘missing and predicted unstable’ from the ‘missing and predicted stable’. Our first principles thermodynamics search includes the examination of (a) the lowest-energy crystalline form of the ABX phase, (b) its stability with respect to decomposition into any combination formed by the A, B and X constituents and (c) the dynamic (phonon) stability of the lowest-energy ternary phase. Note that in search (a) we do not limit the allowed structure to just a single structure type, as in Carrete et al. [18] , where only the cubic LiAlSi-type structure was considered, leading to the elimination of candidate ABX compounds that are stable in other structure types, or in ref. 19 where only the cubic perovskite structural form of ABO 3 were considered for electrocatalysis. Note further that unlike refs 18 , 19 , in step (b) we systematically correct the density-functional values of formation energies [16] , thus avoiding false elimination of stable ternaries on account of the underestimation of their enthalpies. We note that our search is different than ref. 10 where only previously documented oxide materials were examined. Application of first principles thermodynamics based on density-functional methodology [16] , [17] , [20] to a total of 483 ABX compounds (400 missing as well as 83 known [15] ), predicts that the 54 of the 400 missing compounds are stable in specific crystal structures and 346 are predicted unstable. As a test to our thermodynamic equilibrium methodology we apply it to about 30 known (previously synthesized and structurally characterized) ABX compounds listed in ICSD [15] . We find in all cases that these compounds are predicted to be stable in the observed crystal structures, validating the methodology. In the following, we apply the design principles developed above to the stable members of the predicted group of missing ABX compounds and find, contrary to common chemical expectations, that a material made of high atomic number elements can be an insulator and that it tolerates sufficient level of off-stoichiometry to create free holes that avoid the ionic sites and thus can lead to high mobility. Laboratory synthesis then finds TaIrGe to be stable in the predicted crystal structure and p -type transparent conductor with measured large band gap and remarkably high hole mobility of 2,730 cm 2 V −1 s −1 at room temperature. This ‘closure of the loop’ between functionality directed material theory and experiment establishes the promising methodology whereby one first states the target functionality and then looks for the materials having it (‘Inverse Design’). 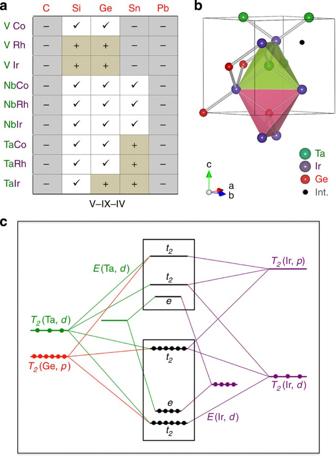Figure 1: Crystal structure and orbital diagram of TaIrGe. (a) ABX compounds in V–IX–IV group. The compounds labelled by check marks (✓) are documented, the compounds marked by plus (+) are predicted stable, and the ones marked by minus (−) are unstable. (b) The stable crystal structure (LiAlSi type, space group: F-43m) of TaIrGe. The small black sphere (indexed as Int.) indicates the empty interstitial site that is equivalent to the Ir site. Two polyhedrons are shown to illustrate the similarity of first shell coordination environment (Ir4tetrahedron) of Ta and Ge. (c) Orbital diagram of TaIrGe as an example of 18-electron ABX half-Heuslers. Design-principle guided search of bulk properties of crystals Figure 1a provides the calculated results on one such group V–IX–IV of 18-electron ABX compounds, with ‘check marks’ indicating previously known compounds, plus signs (+) indicating previously missing and now predicted stable, and minus signs (-) indicate previously missing and now predicted unstable compounds. We next illustrate how a specific functionality is searched. Figure 1: Crystal structure and orbital diagram of TaIrGe. ( a ) ABX compounds in V–IX–IV group. The compounds labelled by check marks ( ✓ ) are documented, the compounds marked by plus (+) are predicted stable, and the ones marked by minus (−) are unstable. ( b ) The stable crystal structure (LiAlSi type, space group: F-43m) of TaIrGe. The small black sphere (indexed as Int.) indicates the empty interstitial site that is equivalent to the Ir site. Two polyhedrons are shown to illustrate the similarity of first shell coordination environment (Ir 4 tetrahedron) of Ta and Ge. ( c ) Orbital diagram of TaIrGe as an example of 18-electron ABX half-Heuslers. Full size image Having supplemented the currently known groups of 18-electron ABX compounds by the previously missing and now predicted stable compounds, we next examine their systematic electronic properties using self-consistent hybrid functional (hybrid exchange–correlation functional (HSE06)) [21] wavefunctions considering the design metrics for p -type transparent conductors. We find a number of new structure–property relationships in this family, which focused our attention to specific subgroups for predicting p -type transparent conductors. First, we find that all 18-electron cubic half-Heusler ABX compounds containing two transition metal atoms (for example, TaIrSn and ZrIrSb), have a band gap between occupied and unoccupied bands (that is, non metals), whereas the cubic 18-electron half-Heusler compounds with one transition metal atom (for example, AlNiP) are metals (see Supplementary Figs 3 and 4 ). Thus, to look for candidate transparent materials we focus on the former group containing two transition elements. The finite band gap in the former case is explained by the strong d – d hybridization between the two transition metals (for example, Ta and Ir) that are nearest neighbour atoms in the half-Heusler (LiAlSi type) structure ( Fig. 1b ), as illustrated for TaIrGe in Fig. 1c . Second, we find that the ABX compounds with heavy X atom tend to be stable in cubic half-Heusler structures; hence can potentially have wide band gaps. For example, the predicted ABX compounds in groups IV–X–IV, IV–IX–V and V–IX–IV with heavy X elements Sb, Bi, Sn or Pb are all stable in cubic structure. In contrast, we find that ABX with light X atoms (that is, O, S, Se, N, P, As, C, Si and Ge) tends to have non-cubic structure and thus are often metallic. This is so because for light X the A and B metals carry ionic charges and thus strongly repel each other when they are nearest neighbours as in the LiAlSi-type structure. We thus look for TCs in heavy X atom compounds. In accordance with the above two structure–property relationships, we identify nine wide gap members in the groups of cubic, two transition element half-Heusler ABX compounds: from the IV–IX–V group we find TiCoSb, TiRhSb, TiIrSb, ZrRhSb, ZrIrSb and HfCoSb; from the IV–X–IV group we find HfPtSn, whereas from the V–IX–IV group we identify TaIrGe and TaIrSn. These are heavy, all-metal atom half-Heusler insulators, in sharp contrast with that many heavy atom compounds tend to be narrow gap semiconductors [22] or semimetals [23] (for example, HgTe, PbSe, PbTe, Bi 2 Se 3 and InSb). The fundamental band gaps of the above nine half-Heuslers are indirect (as illustrated for TaIrGe in Fig. 2a ). Among them, TiIrSb, ZrIrSb, TaIrGe and TaIrSn are newly predicted never before synthesized compounds ( Supplementary Note 1 ). 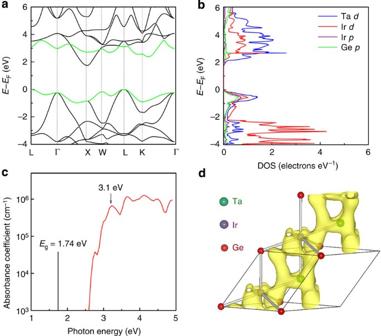Figure 2: Electronic structure and optical properties of TaIrGe. (a) Band structure of TaIrGe. The two approximately parallel valence and conduction bands are highlighted by green giving a gap around 3.1 eV. (b) Angular momentum and site decomposed partial density of states in TaIrGe. (c) Calculated optical absorption coefficient. The black vertical line indicates the predicted minimum band gap. (d) Wavefunction square of the VBM state located at L valley in TaIrGe (isosurface at). Figure 2: Electronic structure and optical properties of TaIrGe. ( a ) Band structure of TaIrGe. The two approximately parallel valence and conduction bands are highlighted by green giving a gap around 3.1 eV. ( b ) Angular momentum and site decomposed partial density of states in TaIrGe. ( c ) Calculated optical absorption coefficient. The black vertical line indicates the predicted minimum band gap. ( d ) Wavefunction square of the VBM state located at L valley in TaIrGe (isosurface at ). Full size image Thermodynamic stability of the heavy, metal atom insulators We evaluate the range of thermodynamic stability of the A–B–X compound as a function of the chemical potentials of A, B and X, considering competing phases composed of the elemental, binary and ternary constituents ( Supplementary Note 2 ). The resulting chemical potential ranges define the thermodynamic growth conditions, which can be used as a guide for experimental synthesis. For the newly predicted and never before synthesized ABX compounds (TiIrSb, ZrIrSb, TaIrGe and TaIrSn), we find that the preferred stability range is located around the boundary of X-richest and A/B-poor growth condition. We next focus on TaIrGe, which has the widest direct band gap and is the only cubic Germanide in the 18-electron ABX family ( Supplementary Note 1 ) Electronic structure and optical transparency The predicted lowest-energy crystal structure of TaIrGe is shown in Fig. 1b . In this structure, both the A and X atoms have B 4 tetrahedrally coordinated environments, and the B atoms are eightfold coordinated by four A atoms and four X atoms. Note the empty interstitial site (as shown by the small black sphere in Fig. 1b ) having the same local environment (that is, A 4 and X 4 tetrahedrons) as the B atoms. Since, all atomic sites have the T d symmetry, the atomic p and d orbitals occur in the solid in the T 2 and E representations of the T d point group. As illustrated in Fig. 1c (see also calculated density of states in Fig. 2b ), the T 2 (Ta, d ) state strongly couples with the T 2 (Ir, d ), state whereas the E (Ta, d ) state couples with E (Ir, d ) state. This pattern of interaction in the cubic structure having two transition metal atoms is responsible for opening a large band gap between the anti-bonding and bonding states. According to our electronic calculation ( Supplementary Note 1 ), this compound has an indirect fundamental band gap of 1.74 eV. The valence band maximum (VBM) and conduction band minimum (CBM) are located the at L valley and X valley, respectively; the smallest direct energy gap between the VB and the CB is at the X valley and has the calculated magnitude of 2.64 eV ( Fig. 2a ). The calculated optical absorption coefficient of TaIrGe based on the GW approximation (Where G stands for Green's Function and W for Coulomb Interaction) [24] for electron’s self-energy is presented in Fig. 2c , showing an optical transition onset at 2.64 eV. Thus TaIrGe is transparent for most visible light. The first strong absorption peak appears at 3.1 eV corresponding to the majority optical transition between the two parallel bands highlighted by green in Fig. 2a . The calculated absorption coefficient has a magnitude of <10 5 cm −1 for photon energy in the range of 2.64–2.9 eV, which is acceptable for thin film transparent conductors. The nature of the hole orbitals promises good carrier mobility Three factors related to the expected intrinsic mobility are noteworthy: First, the hole wavefunction ( Fig. 2d ) is delocalized along the empty interstitial channels (in between the Ta–Ir and the Ta–Ge atoms); this wavefunction pattern avoids the ionic sites that consequently have but a low probability to scatter the mobile carriers. Second, there are quite a few hole states in close energetic proximity to each other, so the effective degeneracy of the hole states in the three-dimensional (3D) momentum space is rather high. For example, the single Γ valley (with threefold band degeneracy per valley) and the sixfold W valley (with single band per valley) lie energetically just below the fourfold L valley (with twofold band degeneracy per valley). Third, whereas conventional oxide transparent conductors generally have rather heavy hole effective mass (because the oxygen-dominated hole states are poorly hybridized) [10] , in a Germanide compound the electron and hole effective masses can be rather low on account of effective hybridization described above. The calculated electron effective masses of TaIrGe, (occurring near the CBM at the X point) are and , and the heavy-hole (HH) and light-hole (LH) effective masses (occurring near the VBM at the L point) are , and , , respectively. All the hole effective masses are significantly lower than those of the conventional p -type transparent oxides [10] , such as CuAlO 2 and SrCu 2 O 2 , which have hole effective masses >2. Design-principle guided search of p -typeness Having identified via functionality-directed discovery an interesting candidate TC material with acceptably large band gaps and consequent optical transparency, we next follow the crucial design principle for p -typeness: screen materials that promote hole-producing defects but suppress hole killers. Our first principles calculations focused on two key quantities for defects: (i) the defect formation energy Δ H ( q , E F , { μ }), which is a function of the defect charge state q , the Fermi-energy E F and the chemical potential { μ } of atoms involved in forming the defect (reflecting the growth conditions) and (ii) the defect charge transition energy (donor or acceptor levels), ɛ ( q/q ′), defined as the E F where the Δ H of a defect at two different charge states q and q ′ are equal. Taking into account Δ H for all intrinsic defects, one can determine the thermodynamic equilibrium Fermi energy E F (eq) ( Figs 3 and 4a ) and the carrier concentration predicted at a given temperature and chemical potential ( Fig. 4b ). 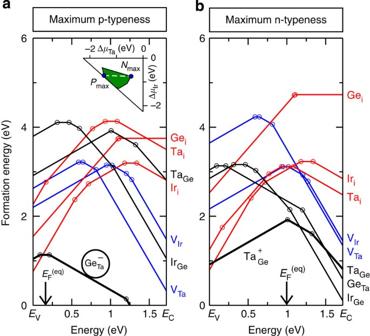Figure 3: Formation energy of selected intrinsic defects of TaIrGe. The energetics are calculated as a function of Fermi levelEFat the chemical condition (ΔμTa, ΔμIr, ΔμGe) that yields the highestp-type carrier concentration,Pmax(a) and that yields the highestn-type carrier concentration,Nmax(b) within the stability triangle (inset ofa). Figure 3: Formation energy of selected intrinsic defects of TaIrGe. The energetics are calculated as a function of Fermi level E F at the chemical condition (Δ μ Ta , Δ μ Ir , Δ μ Ge ) that yields the highest p -type carrier concentration, P max ( a ) and that yields the highest n -type carrier concentration, N max ( b ) within the stability triangle (inset of a ). 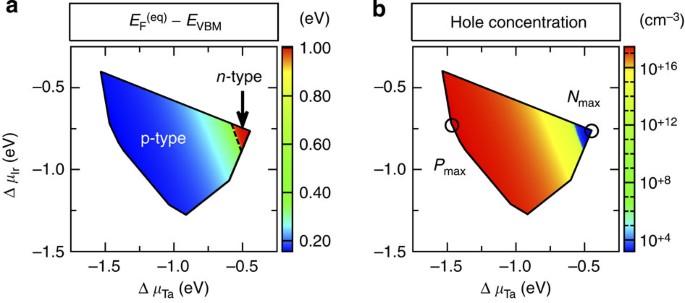Figure 4: Predominance ofp-typeness in TaIrGe across the allowed chemical stability field. (a) Equilibrium Fermi level relative to VBM and (b) intrinsic hole carrier concentration due to intrinsic defects (see e.g. Figure 3). The simulation takes over an initial temperature of 1,200 K, then quenches to room temperature. The excess chemical potential of Ge (ΔμGe) used in defect calculation is determined by the formation enthalpy of TaIrGe ΔHf(TaIrGe)=−0.75 eV per atom, ΔμTaand ΔμIr. The competing phases are shown inSupplementary Table 2. Full size image Figure 4: Predominance of p -typeness in TaIrGe across the allowed chemical stability field. ( a ) Equilibrium Fermi level relative to VBM and ( b ) intrinsic hole carrier concentration due to intrinsic defects (see e.g. Figure 3). The simulation takes over an initial temperature of 1,200 K, then quenches to room temperature. The excess chemical potential of Ge (Δ μ Ge ) used in defect calculation is determined by the formation enthalpy of TaIrGe Δ H f (TaIrGe)=−0.75 eV per atom, Δ μ Ta and Δ μ Ir . The competing phases are shown in Supplementary Table 2 . Full size image Identification of the intrinsic hole producers A most exciting prediction from our intrinsic defect simulation is that TaIrGe displays a strong p -type behaviour ( n hole >10 16 cm −3 , E F (eq) < E VBM +0.2 eV) in the majority of its stability area (bright blue colour in Fig. 4a and bright red colour in Fig. 4b ). From the simulation for crystal growth condition (evaluated at 1,200 K followed by a quench to room temperature), we find the maximum hole concentration of ∼ 2.5 × 10 17 cm −3 at the chemical potential corner labelled P max in the stability area (the most Ta-poor and Ge-rich condition in Fig. 4b ). The hole concentration could be further increased by introducing extrinsic dopants into TaIrGe. The microscopic origin for p -type is revealed by inspecting formation energies of leading defects under the optimal P max chemical potential conditions (inset in Fig. 3a ) (conducive to holes ( p -type)) and as compared with those under the N max condition (conducive to electrons ( n -type)). Out of the 12 intrinsic point defects, including three vacancies (V Ta , V Ir and V Ge ), three interstitials (Ta i , Ir i and Ge i ), and six antisite defects (Ta Ir , Ir Ge , Ir Ge , Ge Ir , Ta Ge and Ge Ta ), we identified Ge-on-Ta antisite defect in (1−) charge state as the dominant acceptor, having lower formation energy than other defects at the Ta-poor conditions ( P max , Fig. 3a ). This acceptor state is derived from the unfilled shallow Ge-4 p state at the Ta-site forming chemical bonds with its nearest neighbour Ir 6 p and 5 d orbitals. The neutral to (1−) charge state transition in Ge Ta occurs at E v+0.21 eV. Considering the 1.74 eV band gap, this transition level is rather close to the VBM. Importantly,the holes produced by Ge Ta 1− are not compensated by the potential hole-killer defects (that is, metal interstitials), that have much higher formation energies ( Fig. 3a ). Laboratory synthesis and crystal structure determination Experimental realization of the hitherto missing (unreported) TaIrGe is accomplished by bulk synthesis methods, followed by optical and electronic characterization. The TaIrGe specimens are synthesized by vacuum annealing the stoichiometric mixture of pure elements (see details in Supplementary Note 3 ). 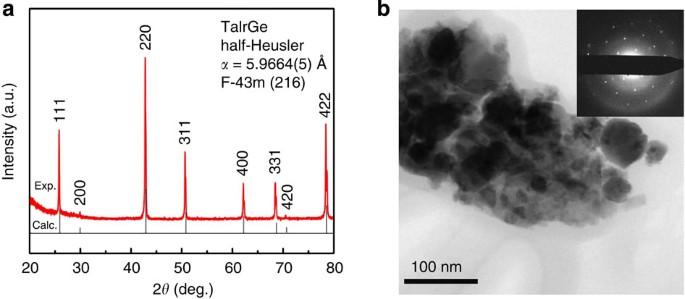Figure 5: Measured crystal structure of TaIrGe. (a) Calculated and experimental XRD pattern of TaIrGe semiconductor. The final phase crystal structure, refined lattice constant, space group and space group number are shown. (b) Representative bright field TEM image of TaIrGe. Inset shows a SAED pattern along at a 110-electron incidence displaying the single crystal nature of the individual grains. Figure 5a shows the X-ray diffraction pattern of TaIrGe, confirming that phase-pure bulk TaIrGe is successfully fabricated. Comparing the experimental X-ray pattern with the calculated diffraction pattern we see good agreement in the positions and intensities of the lines. The refined lattice parameter is 5.9664(5) Å corresponding to a density of 13.94 g cm −3 compared with the calculated lattice parameter of 6.026 Å. The lattice parameters are accurately established using high purity silicon as an internal standard. Figure 5b displays a representative bright field transmission electron microscope (TEM) image and corresponding selected area electron diffraction (SAED) pattern, suggesting a grain size of around 100 nm, and with no secondary phase. Figure 5: Measured crystal structure of TaIrGe. ( a ) Calculated and experimental XRD pattern of TaIrGe semiconductor. The final phase crystal structure, refined lattice constant, space group and space group number are shown. ( b ) Representative bright field TEM image of TaIrGe. Inset shows a SAED pattern along at a 110-electron incidence displaying the single crystal nature of the individual grains. Full size image Measured optical properties The optical absorption spectrum of bulk TaIrGe, obtained from the ultraviolet–visible diffuse reflectance measurements ( Fig. 6a and Supplementary Note 3 ) indicates that TaIrGe exhibits two optical absorption thresholds at about 365 and 485 nm in the visible range (which correspond to band gap energies of 3.39 and 2.55 eV, respectively). Subsequent analyses of the diffuse reflectance using the Kubelka–Munk function [25] , [26] , [27] indicated an indirect transition of 1.64 eV ( Fig. 6b ) and a direct transition of 3.36 eV ( Fig. 6c ). The difference between measured direct optical band gap and the predicted values ( ∼ 3.1 eV) is ∼ 0.2 eV. Thus, the absorption window of TaIrGe covers most of the visible solar spectrum ( ∼ 350 to 700 nm). To confirm this optical band gap, we performed high-vacuum thin-film deposition using TaIrGe target in a pulsed laser deposition system and the obtained 30-nm-thick film is transparent in visible light. 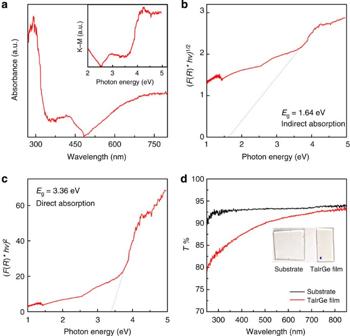Figure 6: Measured optical property of TaIrGe semiconductor. (a) Optical spectra. The absorption spectra are obtained from the ultraviolet/visible diffuse reflectance spectra converted by the Kubelka–Munk26method (arbitrary units). (b,c) The band gap of TaIrGe semiconductor determined by indirect and direct absorption, respectively. The optical band gap is determined by applying Tauc plots34. (d) Transmittence for TaIrGe thin film (∼30 nm thick) grown on Quartz substrate using pulsed laser deposition (PLD) method. The images of the transparent quartz substrate and TaIrGe thin film on substrate are shown in the inset ofd. Figure 6d shows the optical transmittance spectrum of the TaIrGe film grown on transparent quartz substrate, which varies from 85 to 92% in the wavelength region of 350 to 700 nm. This demonstrates that the TaIrGe film is transparent in the visible region. Figure 6: Measured optical property of TaIrGe semiconductor. ( a ) Optical spectra. The absorption spectra are obtained from the ultraviolet/visible diffuse reflectance spectra converted by the Kubelka–Munk [26] method (arbitrary units). ( b , c ) The band gap of TaIrGe semiconductor determined by indirect and direct absorption, respectively. The optical band gap is determined by applying Tauc plots [34] . ( d ) Transmittence for TaIrGe thin film ( ∼ 30 nm thick) grown on Quartz substrate using pulsed laser deposition (PLD) method. The images of the transparent quartz substrate and TaIrGe thin film on substrate are shown in the inset of d . Full size image Measured electrical transport properties The electrical conductivity (σ) of the bulk specimen, measured using Van der Pauw method at room temperature is ∼ 0.35 S cm −1 . The Hall coefficient ( R H ), measured using a five-probe configuration, gave +7.8 × 10 3 cm 3 C −1 , indicative of p -type conduction, which is in agreement with the results from the intrinsic defect calculation. (A Seebeck coefficient is found to be +82 μV K −1 at room temperature for the TaIrGe bulk, further confirming that the TaIrGe is a p -type semiconductor.) Combining the conductivity and Hall coefficient resulted in a hole concentration of ∼ 0.8 × 10 15 cm −3 and a remarkably large Hall mobility of ∼ +2,730 cm 2 V −1 s −1 . The achieved Hall mobility is much higher than that of known p -type transparent conducting oxides [8] , [9] (for example, ∼ 10 cm 2 V −1 s −1 for CuAlO 2 ). We illustrate that a rather rare functionality of p -type transparent conductivity can be discovered by inverse design in a never before made compound. Whereas this functionality has been traditionally searched in the general chemical neighbourhood of compounds containing light element oxides, we use a different search strategy that led to the identification of a good p -type TC in an all-metal heavy atom compound TaIrGe. A remarkable high hole mobility 2,730 cm 2 V −1 s −1 has been found at room temperature. This study opens the way to search transparent conductors among non-oxide heavy-element materials and to designing high-mobility transparent electronic devices. Some of the important insights gained include: Filling the gaps of ‘missing compounds’ in a group of materials allowed a confident formulation of interesting structure–property chemical rules enabling zooming effectively to the subgroup likely to contain p -type TCs. These include the rules that the 18-electron ABX with heavy X atoms tends to have a cubic half-Heusler structure and that insulation band gap are exclusively correlated with the cubic half-Heusler structure having two transition metals. The X-on A antisite hole producer has low formation energy since both A and X sites are in a similar fourfold coordination (whereas B in eightfold) and the size of X (Ge) is smaller than A (Ta). In contrast to the favourable conditions for producing holes, the hole-compensating (electron producing) metal interstitials (Ir i , Ta i and Ge i ) that form by occupying the interstitial site in half-Heusler structure ( Fig. 1b ), require high formation energy due to the large atomic sizes (for Ir i and Ta i ) or repulsion from iso-atom nearest neighbours (for Ta i and Ge i ) and thus do not block the acceptors. The previously studied p -type transparent conductors are prone to have low-hole mobilities [8] , [9] (for example, ∼ 10 cm 2 V −1 s −1 for CuAlO 2 and 0.46 cm 2 V −1 s −1 for SrCu 2 O 2 ), which limited their application. In contrast, the half-Heusler compound TaIrGe can have a hole mobility as high as the standard covalent semiconductor Ge ( ∼ 1,900 cm 2 V −1 s −1 at room temperature [28] ). The electronic structure features that enable good hole mobility include the distribution of the hole VBM wavefunction along interstitial channels that do not pass through ionic sites, the high degeneracy of the hole states in the 3D momentum space near VBM and the relatively low hole effective mass due to significant hybridization ( Fig. 2 ). The proposed approach in inverse design framework starts from the physically formulated design principles of material functionalities, without the preconceived limitations referring to the previous discoveries, considers both existing compounds as well as previously undocumented but now predicted stable members followed by evaluation of design metrics, thereby (significantly) increasing the playing field of discovery, and leads to the efficient selection of candidate materials for experimental realization. This approach, searching directly for specific target functionality (rather than making all compounds at the outset, as in combinatorial synthesis or its computational analogue—high-throughput calculations), as demonstrated in current study, can find interesting candidate materials in unexpected chemical groups of technologically significant functionalities that are hard to find and optimize by rational experiments (for example, p -type TC), potentially opening a new direction to design functional materials (for example, all-heavy-element materials for high-mobility TC). Thermodynamic stability calculations To determine the thermodynamics stability of the ABX compounds, the Δ H f of each ABX compound and all possible competing phases are calculated based on density functional theory (DFT), using the Perdew-Burke-Ernzerhof (PBE) exchange-correlation functional [29] , the projector-augmented wave (PAW) pseudopotential [17] , and the DFT+U method [31] . We use fitted elemental reference energies [16] to correct the DFT error on formation enthalpies (Δ H f ). A compound is considered stable under thermodynamic equilibrium conditions if the values of the chemical potential are such that the formation of a given hypothetical ABX compound is energetically the most favourable of all possible competing phases [17] ( Supplementary Note 2 ). Optical absorption calculations The optical absorption coefficient is calculated using the GW approximation perturbatively on the top of the wavefunctions and energy eigenvalues calculated from a generalized Kohn–Sham scheme with the HSE06 (ref. 21 ) (that is, HSE06+GW, see details in Supplementary Note 1 ). The spin–orbit coupling (SOC) effect in TaIrGe is non-negligible. We calculate the density of states from HSE06 with SOC to compare with that from HSE06 without SOC. The fundamental band gap of TaIrGe is slightly reduced (by <0.1 eV) by SOC ( Supplementary Note 1 ). The electron and hole effective masses are obtained by fitting the actual E – k diagram around CBM and VBM of energy eigenvalues calculated from HSE06, respectively. Defect calculation Defects are calculated in a 2 × 2 × 2 cubic supercell with 96 atoms using the same DFT+U functional as in the thermodynamic stability calculations. The band gap calculated by DFT+U is 1.24 eV, smaller than the GW value 1.74 eV. It is found that from DFT+U to GW, the VBM remains unchanged and CBM undergoes an uplift of 0.5 eV. To correct the finite supercell error, we applied the image charge corrections and band filling corrections as in ref. 32 . A total of 12 types of intrinsic point defects have been calculated, including three vacancies, three interstitial and six antisite defects. We apply the tetrahedral bending mode to the nearest-neighbour atoms [33] . Materials synthesis Polycrystalline TaIrGe samples are synthesized by vacuum annealing a mixture of pure elements in the ratio of 1:1:1 at ∼ 1,200 K for 2 days and quench to room temperature ( Supplementary Note 3 ). X-ray powder diffraction The phase structure of TaIrGe pellets is characterized using a Scintag XDS2000 diffractometer with a Cu-Kα radiation source of wavelength 1.5406, nm operated at 40 kV and 20 mA and a liquid nitrogen-cooled Ge detector (GLP-10195/07-S) over 2 θ angles in the range 20–80°. The lattice parameters are determined using an internal Si standard. The lattice parameters are refined based on whole-pattern fitting Rietveld refinement in the JADE 9.0 software package ( Supplementary Note 3 ). Transmission electron microscope TEM images and SAED pattern are collected on a Hitachi HD-2300A scanning TEM. Optical measurements The ultraviolet–visible diffuse reflectance spectra and transmittance spectrum of the samples are characterized at room temperature in air by a Perkin-Elmer Lambda 1050 UV-Vis/NIR spectrophotometer. Reflectance measurement of the bulk sample is recorded relative to a calibrated standard and the reference material is used to establish a baseline. The diffuse reflectance data are collected in the wavelength range of 250–1,500 nm. Absorption spectra are calculated from the reflectance spectra by means of the standard Kubelka–Munk conversion. The optical band gap is determined from the associated Tauc plots [34] . The transmittance spectrum is determined at room temperature for both the substrate and film. Electrical transport measurement Four-probe resistivity is determined using the Van der Pauw method on the pellet samples by a Physical Measurement System (Quantum Design PPMS 6000). The Seebeck coefficient is obtained from the slope of the thermovoltage versus temperature gradient. The Hall coefficient ( R H ) is measured at room temperature using a five-probe configuration with the magnetic sweep between ±2 T using the PPMS system. How to cite this article: Yan, F. et al. Design and discovery of a novel half-Heusler transparent hole conductor made of all-metallic heavy elements. Nat. Commun. 6:7308 doi: 10.1038/ncomms8308 (2015).